HDAC6 and RhoA are novel players in Abeta-driven disruption of neuronal polarity Maintenance of neuronal polarity and regulation of cytoskeletal dynamics are vital during development and to uphold synaptic activity in neuronal networks. Here we show that soluble β-amyloid (Aβ) disrupts actin and microtubule (MT) dynamics via activation of RhoA and inhibition of histone deacetylase 6 (HDAC6) in cultured hippocampal neurons. The contact of Aβ with the extracellular membrane promotes RhoA activation, leading to growth cone collapse and neurite retraction, which might be responsible for hampered neuronal pathfinding and migration in Alzheimer’s disease (AD). The inhibition of HDAC6 by Aβ increases the level of heterodimeric acetylated tubulin and acetylated tau, both of which have been found altered in AD. We also find that the loss of HDAC6 activity perturbs the integrity of axon initial segment (AIS), resulting in mislocalization of ankyrin G and increased MT instability in the AIS concomitant with loss of polarized localization of tau and impairment of action potential firing. Early deficits in Alzheimer’s disease (AD) are due to neurite degeneration, defects in axonal transport and alterations in the efficiency of neuronal transmission [1] , [2] . In AD, synapse maintenance and reshaping of synaptic contacts are defective and result in early loss of synapses. In neurons, actin filaments are abundant in growth cones and dendritic spines, and disruption of actin turnover results in growth cone collapse [3] . In the mature nervous system, actin filaments form the basis of structural integrity in synapses [4] . On the basis of the critical role of actin in the formation of new synapses and the maintenance of synaptic integrity, we hypothesize that overproduction of beta-amyloid (Aβ) peptide, by inhibiting dynamic changes in actin polymerization, would lead to neurite retraction and synaptic dysfunction. Neurodegenerative stimuli can induce the formation of actin rods [5] where Aβ has been shown to accumulate, and which block transport within neurites [6] . Retracted neurites and disorganized actin filaments are major components of senile plaques and neurofibrillary tangles (NFTs) [7] , which are hallmarks of AD. Aβ and tau are also major components of extracellular senile plaques and intracellular NFTs, respectively, and increasing evidence indicates that the adverse effect of Aβ is dependent on the presence of tau. It has been shown that Aβ is unable to induce neurite degeneration in neurons derived from tau knockout mouse [8] , and that deletion or reduction of endogenous tau prevents the cognitive deficits observed in human amyloid precursor protein transgenic mice [9] . The transport deficit induced by Aβ was also shown to be dependent on tau [10] and exposure of cultured neurons to Aβ leads to missorting of axonal tau into somatodendritic compartments, where it disrupts cytoskeletal components [11] , [12] . Alterations in neuronal polarity can lead not only to functional defects in axon potential propagation but also in the development of young neurons, with dysregulation of adult neurogenesis, a process that is specifically impaired in neurodegenerative diseases. However, the mechanisms and the targets through which Aβ affects cytoskeletal dynamics, and how these may influence axonal elongation or retraction, tau localization and neuronal polarity are still unclear. We exposed neurons both to soluble Aβ 1–42 peptide that is responsible for Aβ-induced toxicity [13] and for the severity of AD [14] , to study MT dynamics, which are crucial in maintaining the integrity of AIS and the axonal localization of tau [15] ; and to beads coated with Aβ to study the direct local effect of extracellular Aβ on actin remodelling, which regulate growth cone movements and axon growth. Recently, tau was demonstrated to be acetylated in the microtubule (MT)-binding domain, a post-translational modification that impairs the binding of tau to MTs, and acetylated tau (ac-tau) was specifically found in tau aggregates in AD and related tauopathies [16] , [17] . Histone deacetylase 6 (HDAC6), a cytosolic member of class II HDACs [18] , is responsible for deacetylating both tubulin [19] and tau [16] . Intriguingly, neurons in which HDAC6 were knocked down lose the axonal initial segment (AIS) [20] , a trafficking barrier important for maintaining the polarized localization of axonal proteins, although the mechanism remains unknown. The maintenance of neuronal polarity depends on the AIS region in which proteins are stabilized and organized by ankyrin G (ankG). In the AIS, MTs are stabilized by the binding of the MT plus-end-binding protein 3 (EB3) to ankG [21] , and HDAC6, as a MT-capping protein, may contribute to MT stability [22] . It is thus important to establish the possible link between the increased acetylation found in AD, the activity of HDAC6 and Aβ. Here we provide evidence that the contact of extracellular Aβ with the plasma membrane is sufficient to induce growth cone collapse by activation of the RhoA/ROCK-dependent pathway and increase in actin retrograde flow in neuronal growth cones, with destructive effect on neurite outgrowth. In addition, we show for the first time that internalized Aβ inhibits HDAC6 inducing an increase in the acetylation of α/β-tubulin heterodimers and of tau. Furthermore, we demonstrate that Aβ increased MT dynamics in the AIS, disrupting the barrier and leading to missorting of tau in minor neurites, effects that are prevented by HDAC6 overexpression. We propose that activation of the RhoA–ROCK pathway by extracellular Aβ and inhibition of HDAC6 by intracellular Aβ result in cytoskeletal instability in neurites and in the AIS, leading to loss of neuronal polarity. Extracellular Aβ induces neurite retraction Neurite outgrowth and retraction are processes tightly regulated by cytoskeletal dynamics. Previous studies reported that Aβ fibrils reduce neurite outgrowth via activation of RhoA in a neuroblastoma cell line [23] and in hippocampal neurons [24] . Aβ is released extracellularly on cleavage of amyloid precursor protein at the plasma membrane or in endosomes, and the monomeric form is present in the extracellular milieu before aggregation might take place. To investigate whether Aβ is able to influence axonal elongation, we used the purified soluble form of Aβ. Its molecular state was assessed by western blot and atomic force microscopy (AFM) ( Supplementary Fig. 1a,b ) showing that Aβ was mostly in the monomeric form and few oligomers were present after 1-h incubation in neuronal medium. Embryonic hippocampal neurons at 3 days in vitro (DIV) were incubated with 1 μM Aβ for 1 h and the length of axons was measured by axonal tracing. In the presence of Aβ, the average axonal length was decreased by 31.7% of control axons ( Fig. 1a ). The longest neurite was considered as axon, as demonstrated by the polarized localization of tau ( Fig. 1b ). The average growth of 3 DIV hippocampal neurons in our conditions was of ∼ 20 μm h −1 . The length of the axon in neurons incubated with Aβ for 1 h was ∼ 35 μm shorter with respect to that of control neurons and was therefore suggestive of axonal retraction. To better understand the mechanism underlying retraction of the specific neurite under the influence of extracellular Aβ, we used optically driven Aβ- or scrambled Aβ-coated microspheres brought in contact with the neck of axonal growth cone ( Fig. 1c ). Coating of microspheres was verified by confocal imaging ( Fig. 1d ), and the local application of Aβ bound to microspheres induced growth cone collapse, as indicated by a 52.9% reduction in the growth cone surface area after 30 min ( Fig. 1e ), with complete collapse after 40 min. The effect of Aβ was prevented by the inhibitor of Rho-associated kinase (ROCK) Y27632, and by the myosin II inhibitor, blebbistatin, indicating the involvement of ROCK-dependent pathway and actin retrograde flow in the collapse of the growth cone ( Fig. 1c,e ). 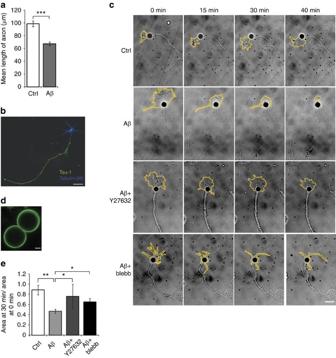Figure 1: Extracellular Aβ induces neurite retraction via ROCK-dependent pathway. (a) Bar graph showing the mean axonal length of neurons incubated either with 0.05% DMSO (ctrl, 98.79±4.44,n=134) or with 1 μM Aβ (Aβ, 67.51±2.77,n=159) for 1 h, measured by axon tracing. Statistical significance determined by two-tailedt-test, **P<0.001. (b) Fluorescence analysis of tau (green) and tubulin-βIII (blue) localization in cultured hippocampal neuron at 3 DIV, showing tau polarization in axons. Scale bar, 25 μm. (c) Images taken at 0, 15, 30 and 40 min from time-lapse movies of embryonic hippocampal neurons in the presence of optically driven microspheres coated with scrambled Aβ (top panels), Aβ (middle panels), with Aβ and 10 μM Y27632, a ROCK inhibitor (lower panels), or with Aβ and 10 μM blebbistatin, a myosin II inhibitor. The growth cone area (highlighted in yellow) shows a reduction upon contact with the Aβ-coated microsphere that is prevented by Y27632 and by blebbistatin. Scale bar, 25 μm. (d) Confocal image showing successful coating of microspheres with fluorescently labelled Aβ peptide. Scale bar, 1 μm. (e) Bar graph showing the ratio between the growth cone area at the end and that at the start of time-lapse movies as inc. Scrambled Aβ (ctrl, 1.05±0.11,n=6), Aβ (Aβ, 0.43±0.04,n=7), Aβ+10 μM Y27632 (Aβ +Y27632, 0.93±0.24,n=4) and Aβ+10 μM blebbistatin (Aβ+blebb, 0.70±0.07,n=3). Statistical significance determined by two-tailedt-test, **P<0.001 (ctrl/Aβ), *P=0.034 (Aβ/Aβ +Y27632), *P=0.009 (Aβ/Aβ+blebb). Inaande, data are expressed as mean±s.e.m. Figure 1: Extracellular Aβ induces neurite retraction via ROCK-dependent pathway. ( a ) Bar graph showing the mean axonal length of neurons incubated either with 0.05% DMSO (ctrl, 98.79±4.44, n =134) or with 1 μM Aβ (Aβ, 67.51±2.77, n =159) for 1 h, measured by axon tracing. Statistical significance determined by two-tailed t -test, ** P <0.001. ( b ) Fluorescence analysis of tau (green) and tubulin-βIII (blue) localization in cultured hippocampal neuron at 3 DIV, showing tau polarization in axons. Scale bar, 25 μm. ( c ) Images taken at 0, 15, 30 and 40 min from time-lapse movies of embryonic hippocampal neurons in the presence of optically driven microspheres coated with scrambled Aβ (top panels), Aβ (middle panels), with Aβ and 10 μM Y27632, a ROCK inhibitor (lower panels), or with Aβ and 10 μM blebbistatin, a myosin II inhibitor. The growth cone area (highlighted in yellow) shows a reduction upon contact with the Aβ-coated microsphere that is prevented by Y27632 and by blebbistatin. Scale bar, 25 μm. ( d ) Confocal image showing successful coating of microspheres with fluorescently labelled Aβ peptide. Scale bar, 1 μm. ( e ) Bar graph showing the ratio between the growth cone area at the end and that at the start of time-lapse movies as in c . Scrambled Aβ (ctrl, 1.05±0.11, n =6), Aβ (Aβ, 0.43±0.04, n =7), Aβ+10 μM Y27632 (Aβ +Y27632, 0.93±0.24, n =4) and Aβ+10 μM blebbistatin (Aβ+blebb, 0.70±0.07, n =3). Statistical significance determined by two-tailed t -test, ** P <0.001 (ctrl/Aβ), * P =0.034 (Aβ/Aβ +Y27632), * P =0.009 (Aβ/Aβ+blebb). In a and e , data are expressed as mean±s.e.m. Full size image Extracellular Aβ alters growth cone adhesion and motility To monitor cytoskeletal dynamics in the axonal growth cone throughout the external local application of Aβ-coated microspheres, we performed simultaneous bright-field imaging of the neuron and force spectroscopy measurement on the adhered coated microsphere positioned on the neck of the growth cone ( Supplementary Fig. 2a ). The movement of the microsphere, measured through a force-clamp system [25] , is dissected in two distinct components ( Supplementary Fig. 2b and Methods section). The low-frequency component of the motion is associated with the cytoskeletal dynamics underlying the remodelling of the membrane-leading edge, and it is recorded through the PIEZO stage, which tracks the bead position ( Supplementary Fig. 2c , upper panel). The high-frequency component of the motion, representing the Brownian fluctuation of the bead, is associated with the strength of the adhesion between the bead and the cell membrane, and is measured by the quadrant photodiode (QPD) ( Supplementary Fig. 2c , lower panel). The variance of the QPD signal decreases when the adhesion contact is stabilized through the binding to a receptor, or by receptors clustering at the bead contact. The low- and high-frequency components of the bead motion are prevalently influenced by actin polymerization [26] , [27] and myosin II motor contraction [28] . The change in the variance associated with the presence of the bead could be biased on the presence of previously established focal adhesions at the contact point that strongly influence the local cytoskeletal organization. In our experimental conditions, the bead was attached to the apical surface, where two-dimensional cultured cells are normally unable to establish adhesion structures, due to the lack of mechanical constraint. Therefore, the bead positioned on the surface of the growth cone can be considered the first and only mechanical constraint experienced by the cell. Correspondingly, the observed dynamics are associated with the formation of an adhesion contact caught at its onset, in a reproducible way between all neurons examined. Application of Aβ-coated microspheres induced a large and fast decrease in the variance with respect to control that was prevented by cell treatment with Y27632 or blebbistatin ( Supplementary Fig. 2d ; Fig. 2a ), suggesting that in the presence of Aβ, the tightening of the adhesion with the membrane is faster and stronger, and involves activation of ROCK. To quantify Aβ-induced growth cone collapse ( Fig. 1e ), we monitored the vertical position Sz of the bead as a function of time ( Supplementary Fig. 2e ). The bead was attached at the neck of the growth cone, and, with Aβ-coated microspheres, the height of the bead decreased by ∼ 2 μm in 45 min, due to emptying of the growth cone content that subsequently leads to axon shrinking, while with scrambled Aβ-coated microsphere, we observed fluctuation of the bead height in the range of few hundred nanometres, not associated with decrease in thickness of the growth cone neck. The shrinking effect induced by Aβ-coated microspheres was prevented by incubation of neurons with Y27632 or blebbistatin ( Fig. 2b ). Similar difference between Aβ and control appeared when we looked at the average microsphere velocity, an index of active reshaping of the cell associated with cytoskeleton dynamics ( Supplementary Fig. 2f ). The normalized cumulative histogram of the microsphere velocity ( Fig. 2c ) shows that with Aβ-coated microspheres (in red) the curve is clearly shifted towards zero, indicating impaired assembly and disassembly of cytoskeletal filaments. The treatment with Y27632 or blebbistatin partially prevented the inhibition of cell reshaping due to Aβ. 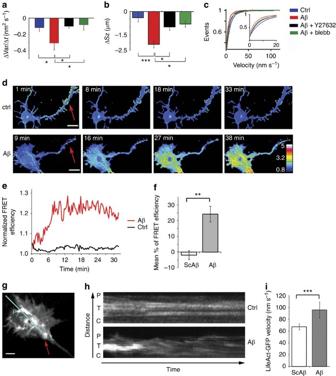Figure 2: Extracellular Aβ alters cytoskeleton dynamics by activating RhoA and increases F-actin retrograde flow. (a) Quantification of the Brownian motion variance decrease. Scrambled Aβ (blue, −0.15±0.05,n=8); Aβ (red, −0.31±0.08,n=9); Aβ+blebb (green, −0.08±0.06,n=5); and Aβ+Y27632 (black, −0.1±0.02,n=5). Statistical significance determined by one-way ANOVA,*P=0.034 (ctrl/Aβ), *P=0.035 (Aβ/Aβ-Y27632), *P=0.033 (Aβ/Aβ-blebb). (b) Quantification of the decrease in thezcoordinate. Scrambled Aβ (blue, −0.4±0.26); Aβ (red, −2.11±0.21); Aβ+blebb (green, −0.8±0.18); and Aβ+Y27632 (black, −1.1±0.19).nas ina. Statistical significance determined by one-way ANOVA, ***P<0.001 (ctrl/Aβ), *P=0.028 (Aβ/Aβ+Y27632), *P=0.012 (Aβ/Aβ+blebb). (c) Normalized cumulative histograms of the microsphere velocity. An enlargement is shown in the inset. Statistical significance determined by two sample Kolmogorov–Smirnov test,P<10−26(ctrl/Aβ),P=0.002 (Aβ/Aβ+blebb),P<10−8(Aβ/Aβ+Y27632),P=0.002 (ctrl/Aβ+Y27632),P<10−28(ctrl/Aβ+blebb),P=0.04 (Aβ+blebb/Aβ+Y27632). (d) Images of YFP/CFP ratio in neurons overexpressing the FRET probe Raichu-RhoA. A scrambled Aβ (top panels) or Aβ (bottom panels)-coated microsphere was attached to the neurite (red arrows). A pseudocoloured scale of the YFP/CFP ratio is shown in the lower right image. Scale bars: upper row, 12 μm; lower row, 10 μm. (e) Representative curves of the normalized FRET efficiency in neurons overexpressing Raichu-RhoA and treated as ind. Scrambled Aβ (black) and Aβ (red). (f) Quantification of FRET efficiency in the neurite of neurons treated as ind. Scrambled Aβ (ctrl, −1.93±2.85,n=6) and Aβ (Aβ, 24.21±4.93,n=10). Statistical significance determined by two-tailedt-test, **P=0.0018. (g) Example of a neuron electroporated with LifeAct-GFP and put in contact with a microsphere (red arrow). Kymographs were constructed along the light blue line. Scale bar, 5 μm. (h) Representative kymographs obtained from time-lapse movies of LifeAct-GFP-electroporated neurons in the presence of scrambled Aβ- (ctrl, top panel) or Aβ-coated microspheres (Aβ, bottom panel). Ingandh, peripheral domain (P), transition zone (T) and central domain (C). (i) Quantification of LifeAct-GFP velocity obtained from kymographs as inh. Scrambled Aβ (Sc Aβ, 67.70±3.91, slopesn=54) and Aβ (Aβ, 92.95±6.51, slopesn=49). Statistical significance determined by two-tailedt-test, ***P=0.001. Ina,b,fandi, data are expressed as mean±s.e.m. ANOVA, analysis of variance. Figure 2: Extracellular Aβ alters cytoskeleton dynamics by activating RhoA and increases F-actin retrograde flow. ( a ) Quantification of the Brownian motion variance decrease. Scrambled Aβ (blue, −0.15±0.05, n =8); Aβ (red, −0.31±0.08, n =9); Aβ+blebb (green, −0.08±0.06, n =5); and Aβ+Y27632 (black, −0.1±0.02, n =5). Statistical significance determined by one-way ANOVA,* P =0.034 (ctrl/Aβ), * P =0.035 (Aβ/Aβ-Y27632), * P =0.033 (Aβ/Aβ-blebb). ( b ) Quantification of the decrease in the z coordinate. Scrambled Aβ (blue, −0.4±0.26); Aβ (red, −2.11±0.21); Aβ+blebb (green, −0.8±0.18); and Aβ+Y27632 (black, −1.1±0.19). n as in a . Statistical significance determined by one-way ANOVA, *** P <0.001 (ctrl/Aβ), * P =0.028 (Aβ/Aβ+Y27632), * P =0.012 (Aβ/Aβ+blebb). ( c ) Normalized cumulative histograms of the microsphere velocity. An enlargement is shown in the inset. Statistical significance determined by two sample Kolmogorov–Smirnov test, P <10 −26 (ctrl/Aβ), P =0.002 (Aβ/Aβ+blebb), P <10 −8 (Aβ/Aβ+Y27632), P =0.002 (ctrl/Aβ+Y27632), P <10 −28 (ctrl/Aβ+blebb), P =0.04 (Aβ+blebb/Aβ+Y27632). ( d ) Images of YFP/CFP ratio in neurons overexpressing the FRET probe Raichu-RhoA. A scrambled Aβ (top panels) or Aβ (bottom panels)-coated microsphere was attached to the neurite (red arrows). A pseudocoloured scale of the YFP/CFP ratio is shown in the lower right image. Scale bars: upper row, 12 μm; lower row, 10 μm. ( e ) Representative curves of the normalized FRET efficiency in neurons overexpressing Raichu-RhoA and treated as in d . Scrambled Aβ (black) and Aβ (red). ( f ) Quantification of FRET efficiency in the neurite of neurons treated as in d . Scrambled Aβ (ctrl, −1.93±2.85, n =6) and Aβ (Aβ, 24.21±4.93, n =10). Statistical significance determined by two-tailed t -test, ** P =0.0018. ( g ) Example of a neuron electroporated with LifeAct-GFP and put in contact with a microsphere (red arrow). Kymographs were constructed along the light blue line. Scale bar, 5 μm. ( h ) Representative kymographs obtained from time-lapse movies of LifeAct-GFP-electroporated neurons in the presence of scrambled Aβ- (ctrl, top panel) or Aβ-coated microspheres (Aβ, bottom panel). In g and h , peripheral domain (P), transition zone (T) and central domain (C). ( i ) Quantification of LifeAct-GFP velocity obtained from kymographs as in h . Scrambled Aβ (Sc Aβ, 67.70±3.91, slopes n =54) and Aβ (Aβ, 92.95±6.51, slopes n =49). Statistical significance determined by two-tailed t -test, *** P =0.001. In a , b , f and i , data are expressed as mean±s.e.m. ANOVA, analysis of variance. Full size image Taken together, these results suggest that axon retraction is induced by increased myosin II-mediated actin retrograde flow, with ensuing substantial and fast stabilization of cell–microsphere adhesion contact. Furthermore, the similarity in the velocity distribution obtained with Y27632 or blebbistatin suggests that ROCK and myosin II are part of the same pathway affected by local delivery of Aβ on the neuronal surface. Extracellular Aβ increases actin retrograde flow The involvement of ROCK and myosin II in Aβ-driven growth cone collapse was suggestive of the activation of RhoA, whose downstream target is ROCK. We took advantage of the intramolecular fluorescence-resonance energy transfer (FRET) probe Raichu, a biosensor of RhoA activity [29] , to follow the localized activation of RhoA in the presence of Aβ-coated microspheres, optically driven in contact with the distal part of the axon of cultured neurons ( Fig. 2d ). Images in the YFP and CFP emission wavelengths were acquired separately for 30 min and FRET efficiency was calculated as acceptor/donor ratio ( Fig. 2e ). The contact with Aβ-coated microsphere induced a 24% increase in FRET efficiency compared with that in control neurons (in contact with scrambled Aβ-coated microsphere) ( Fig. 2f ). To confirm the activation of RhoA, which is known to regulate actin retrograde flow, actomyosin contraction was evaluated in the presence of Aβ-coated microspheres. Neurons were electroporated with LifeAct-green fluorescent protein (GFP), to follow the movement of microfilaments, to which LifeAct specifically binds. Kymographs were assembled from live-imaging movies of the growth cone ( Fig. 2g ) to measure the rate of actin retrograde flow in the presence of Aβ-coated or scrambled Aβ-coated microspheres ( Fig. 2h ). Statistical analysis demonstrated a significant ∼ 40% increase of actin retrograde flow induced by extracellular Aβ compared with scrambled Aβ ( Fig. 2i ), suggesting that actin retrograde flow might be responsible for the observed growth cone collapse in neurons exposed to Aβ. Aβ increases MT dynamics and increases acetylated tubulin RhoA activation has been previously shown to stabilize MT [30] , which show long half-life and result capped at their plus end. Post-translational modifications of MT, such as acetylation and detyrosination, or tyrosination have been studied as markers for stabilized MT or for dynamic MT, respectively [31] . We therefore analysed the levels of acetylated tubulin (ac-tub) by immunofluorescent staining of neurons exposed or not to Aβ. An increase in ac-tub was evident after 1 h of exposure to Aβ and quantified as ∼ 30% higher than in control, while tubulin-βIII showed no change. Taxol, a MT stabilizer, and tubacin, a specific inhibitor of HDAC6 deacetylase, were used as positive controls and induced an increase of ∼ 50 and ∼ 40%, respectively, of the signal of ac-tub ( Fig. 3a,b ). RhoA activation by Aβ and stabilization of MT would also result in inhibition of MT dynamics [32] . To determine MT dynamics, we analysed the rate of movement of the fluorescent comets of EB3, in neurons overexpressing EB3-GFP on incubation with soluble Aβ by total internal reflection live-imaging microscopy. Surprisingly, we observed that Aβ was able to increase the average speed of EB3-GFP comets by ∼ 40% ( Fig. 3c ), in apparent contradiction with the effect of Aβ on acetylation of MT; however, also in the presence of tubacin, which induced MT acetylation, the speed of EB3 comets was almost doubled. The analysis of Aβ effect on MT was performed after 1-h incubation with the peptide, to allow internalization of Aβ ( Supplementary Fig. 3 ); therefore, the effects of Aβ will result from its action both at the cell membrane and in the intracellular space. 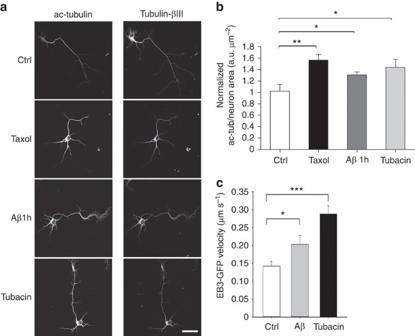Figure 3: Aβ increases the MT plus-end dynamics and acetylated tubulin. (a) Fluorescence analysis of acetylated tubulin (ac-tub) in hippocampal neurons treated with either 0.05% DMSO (ctrl) for 1 h, 1 μM taxol for 30 min, 100 nM Aβ for 1 h or 10 μM tubacin for 1 h showing increased intensity of ac-tub staining in Aβ-, tubacin- and taxol-treated neurons compared with control. Scale bar, 25 μm. (b) Quantification of ac-tub staining intensity normalized to the neuron area calculated from the area of tubulin-βIII immunofluorescence. Hippocampal neurons were treated with either 0.05% DMSO for 1 h (ctrl, 1±0.12,n=24), 1 μM taxol for 30 min (taxol, 1.56±0.10,n=30), 100 nM Aβ for 1 h (Aβ1h, 1.31±0.05,n=31) or 10 μM tubacin for 1 h (tubacin, 1.44±0.14,n=23). Statistical significance determined by one-way ANOVA, **P=0.002 (ctrl versus taxol), *P=0.04 (ctrl versus Aβ), *P=0.02 (ctrl versus tubacin). (c) Bar graph showing the mean speed of GFP comets in EB3-GFP-electroporated neurons, preincubated with 0.05% DMSO (ctrl, 0.14±0.01,n=22), 100 nM Aβ for 1 h (Aβ, 0.20±0.02,n=16) or 10 μM tubacin for 1 h (0.29±0.02,n=6), and imaged for 90 s. Statistical significance determined by one-way ANOVA,*P=0.039, ***P<0.001. Inbandc, data are expressed as mean±s.e.m. ANOVA, analysis of variance. Figure 3: Aβ increases the MT plus-end dynamics and acetylated tubulin. ( a ) Fluorescence analysis of acetylated tubulin (ac-tub) in hippocampal neurons treated with either 0.05% DMSO (ctrl) for 1 h, 1 μM taxol for 30 min, 100 nM Aβ for 1 h or 10 μM tubacin for 1 h showing increased intensity of ac-tub staining in Aβ-, tubacin- and taxol-treated neurons compared with control. Scale bar, 25 μm. ( b ) Quantification of ac-tub staining intensity normalized to the neuron area calculated from the area of tubulin-βIII immunofluorescence. Hippocampal neurons were treated with either 0.05% DMSO for 1 h (ctrl, 1±0.12, n =24), 1 μM taxol for 30 min (taxol, 1.56±0.10, n =30), 100 nM Aβ for 1 h (Aβ1h, 1.31±0.05, n =31) or 10 μM tubacin for 1 h (tubacin, 1.44±0.14, n =23). Statistical significance determined by one-way ANOVA, ** P =0.002 (ctrl versus taxol), * P =0.04 (ctrl versus Aβ), * P =0.02 (ctrl versus tubacin). ( c ) Bar graph showing the mean speed of GFP comets in EB3-GFP-electroporated neurons, preincubated with 0.05% DMSO (ctrl, 0.14±0.01, n =22), 100 nM Aβ for 1 h (Aβ, 0.20±0.02, n =16) or 10 μM tubacin for 1 h (0.29±0.02, n =6), and imaged for 90 s. Statistical significance determined by one-way ANOVA,* P =0.039, *** P <0.001. In b and c , data are expressed as mean±s.e.m. ANOVA, analysis of variance. Full size image Aβ inhibits HDAC6 We therefore wondered whether the increase in acetylation could be due to ac-tub hetereodimers rather than to acetylated MT, as MT were in a more dynamic state in the presence of Aβ, as shown by the measure of EB3 velocity. To address this hypothesis, we performed ac-tub immunostaining after permeabilization of neurons with Tx-100, to induce leakage of heterodimers, keeping only polymerized MT inside the cell. Indeed, in neurons treated with 1 μM taxol and permeabilized, the signal of ac-tub was stronger than that of control, while after 1 h of exposure to Aβ, and similarly after exposure to tubacin, the signal of ac-tub was comparable to that of control neurons ( Fig. 4a,b ). Physiologically, acetylation of tubulin occurs preferentially on polymerized MT [33] , whereas deacetylation of α-tubulin by HDAC6 is thought to occur when α-tubulin is in a heterodimeric state [34] . Therefore, HDAC6 might be a target of Aβ, translating its effect on tubulin acetylation. To measure the catalytic activity of HDAC6, we performed an in vitro assay using purified HDAC6 together with Aβ or the HDAC inhibitor trichostatin A (TSA) as a positive control. Statistical analysis indicated ∼ 25% and ∼ 12% significant inhibition of HDAC6 activity by 1 μM and 100 nM Aβ, respectively, with TSA inducing a ∼ 50% decrease in respect to control ( Fig. 4c ), suggesting direct inhibitory interaction of Aβ with HDAC6, at least in vitro . The increase in ac-tub induced by Aβ was confirmed by western blot analysis. Lysates of neurons treated with Aβ show increase in ac-tub as expected ( Fig. 4d , ac-tub, first two lanes). Analysis of lysates from neurons fixed after the incubation period, to maintain MT and monomers in the original conditions of polymerization, confirmed that exposure of neurons to Aβ induced an increase of ac-tub besides MT, appreciable as a band at 52 kDa and bands at higher molecular weight, respectively, similarly to the effect of exposure to tubacin. Taxol, consistently with the results shown in the immunofluorescence experiment on permeabilized neurons, preferentially induces acetylation of MT ( Fig. 4d , ac-tub, last four lanes; Fig. 4e ). The effect of internalized Aβ, arising at later time points in respect of the one induced by contact with the plasma membrane, appears to be associated with increased MT dynamics. To further examine the action of Aβ on MT, we assessed the number of catastrophes/pauses, finding a significant ∼ 50% increase on incubation with Aβ ( Fig. 4f ), possibly because of the combined action of Aβ on MT and actin retrograde flow, suggesting that MTs are in a highly unstable state after Aβ treatment. 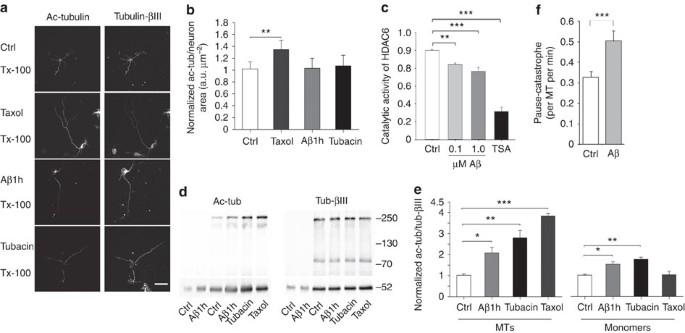Figure 4: Aβ inhibits HDAC6 and increases acetylation of tubulin heterodimers. (a) Fluorescence analysis of ac-tub in neurons treated with either 0.05% DMSO (ctrl) for 1 h, 1 μM taxol for 30 min, 100 nM Aβ for 1 h or 10 μM tubacin for 1 h, and permeabilized. Scale bar, 25 μm. (b) Quantification of ac-tub staining intensity normalized to neuronal area calculated from tubulin-βIII immunofluorescence in permeabilized neurons. Neurons were treated with either 0.05% DMSO for 1 h (ctrl, 1±0.12,n=25), 1 μM taxol for 30 min (1.35±0.15,n=26), 100 nM Aβ for 1 h (Aβ, 1.03±0.17,n=30) or 10 μM tubacin for 1 h (tubacin, 1.07±0.18,n=16). Statistical significance determined by one-way ANOVA, **P=0.035. (c)In vitroassay of the catalytic activity of HDAC6 in the presence of either DMSO (ctrl, 1.00±0.00,n=10), 100 nM Aβ (Aβ 0.1, 0.86±0.02,n=8), 1 μM Aβ (Aβ 1.0, 0.78±0.04,n=8) or 50 nM trichostatin A (TSA, 0.14±0.05,n=10) normalized to the control. Statistical significance determined by one-way ANOVA, **P=0.006, ***P<0.001. (d) Representative immunoblot showing ac-tub and tubulin-βIII in MT (higher bands) and monomers (band at 52 kDa) from lysate of not fixed (first two lanes) or fixed (last four lanes) neurons treated with 0.05% DMSO for 1 h (ctrl), 100 nM Aβ for 1 h (Aβ1h), 10 μM tubacin for 1 h (tubacin) or 1 μM taxol for 30 min (taxol). One out of ten of lysate from non-fixed samples was loaded. (e) Quantification of the ratio between ac-tub and tubulin-βIII levels performed on the sum of the bands above 52 kDa (MTs) and on the band at 52 kDa (monomers) from neurons treated as inaand fixed,n=3. Statistical significance determined by one-way ANOVA. MT: *P=0.04 (ctrl/Aβ1h, 2.08±0.27); **P=0.003 (ctrl/tubacin, 2.80±0.35); ***P<0.001 (ctrl/taxol, 3.84±0.12). Monomers: *P=0.04 (ctrl/Aβ1h, 1.53±0.12); **P=0.004 (ctrl/tubacin, 1.77±0.10); (ctrl/taxol, 1.02±0.18). (f) Bar graph showing the number of pause/catastrophe in neurons electroporated as inFig. 3cand incubated with 0.05% DMSO (ctrl, 0.33±0.03,n=401 from 43 neurons) or 100 nM Aβ (Aβ, 0.50±0.05,n=222 from 28 neurons). Statistical significance determined by two-tailedt-test, ***P<0.001. Inb,c,eandf, data are expressed as mean±s.e.m. ANOVA, analysis of variance. Figure 4: Aβ inhibits HDAC6 and increases acetylation of tubulin heterodimers. ( a ) Fluorescence analysis of ac-tub in neurons treated with either 0.05% DMSO (ctrl) for 1 h, 1 μM taxol for 30 min, 100 nM Aβ for 1 h or 10 μM tubacin for 1 h, and permeabilized. Scale bar, 25 μm. ( b ) Quantification of ac-tub staining intensity normalized to neuronal area calculated from tubulin-βIII immunofluorescence in permeabilized neurons. Neurons were treated with either 0.05% DMSO for 1 h (ctrl, 1±0.12, n =25), 1 μM taxol for 30 min (1.35±0.15, n =26), 100 nM Aβ for 1 h (Aβ, 1.03±0.17, n =30) or 10 μM tubacin for 1 h (tubacin, 1.07±0.18, n =16). Statistical significance determined by one-way ANOVA, ** P =0.035. ( c ) In vitro assay of the catalytic activity of HDAC6 in the presence of either DMSO (ctrl, 1.00±0.00, n =10), 100 nM Aβ (Aβ 0.1, 0.86±0.02, n =8), 1 μM Aβ (Aβ 1.0, 0.78±0.04, n =8) or 50 nM trichostatin A (TSA, 0.14±0.05, n =10) normalized to the control. Statistical significance determined by one-way ANOVA, ** P =0.006, *** P <0.001. ( d ) Representative immunoblot showing ac-tub and tubulin-βIII in MT (higher bands) and monomers (band at 52 kDa) from lysate of not fixed (first two lanes) or fixed (last four lanes) neurons treated with 0.05% DMSO for 1 h (ctrl), 100 nM Aβ for 1 h (Aβ1h), 10 μM tubacin for 1 h (tubacin) or 1 μM taxol for 30 min (taxol). One out of ten of lysate from non-fixed samples was loaded. ( e ) Quantification of the ratio between ac-tub and tubulin-βIII levels performed on the sum of the bands above 52 kDa (MTs) and on the band at 52 kDa (monomers) from neurons treated as in a and fixed, n =3. Statistical significance determined by one-way ANOVA. MT: * P =0.04 (ctrl/Aβ1h, 2.08±0.27); ** P =0.003 (ctrl/tubacin, 2.80±0.35); *** P <0.001 (ctrl/taxol, 3.84±0.12). Monomers: * P =0.04 (ctrl/Aβ1h, 1.53±0.12); ** P =0.004 (ctrl/tubacin, 1.77±0.10); (ctrl/taxol, 1.02±0.18). ( f ) Bar graph showing the number of pause/catastrophe in neurons electroporated as in Fig. 3c and incubated with 0.05% DMSO (ctrl, 0.33±0.03, n =401 from 43 neurons) or 100 nM Aβ (Aβ, 0.50±0.05, n =222 from 28 neurons). Statistical significance determined by two-tailed t -test, *** P <0.001. In b , c , e and f , data are expressed as mean±s.e.m. ANOVA, analysis of variance. Full size image Aβ increases acetylated tau and induces missorting of tau Destabilization of MT in AD pathology is mainly attributed to the dissociation of tau, the main axonal microtubule-associated protein (MAP). In the light of a recent study showing that HDAC6, in addition to SIRT1 (ref. 17 ), also deacetylates tau [16] , we analysed the level of ac-tau on Aβ treatment. After exposure of neurons to 100 nM, or 1 μM Aβ or 100 nM TSA, tau immunoprecipitated from neuronal lysates showed increased acetylation ( Fig. 5a,b ). As acetylation of tau has been shown to correlate with decreased MT-binding capability [16] , which induces disruption of tau retrograde barrier [15] , we analysed tau localization on exposure to Aβ. In 3 DIV neurons treated with 100 nM Aβ, tau-1 staining was present also in minor neurites ( Fig. 5c ) and the percentage of neurons with tau-1 localization restricted to the axon was significantly decreased, being ∼ 2.5-fold less than that of control; inhibition of HDAC6 by tubacin yielded similar results ( Fig. 5d ). Tau missorting was observed both in young neurons at 3 DIV and in neurons at later stage of development (14 DIV) ( Fig. 5c ; Supplementary Fig. 4a ). Neurons were co-electroporated with HDAC6-FLAG together with GFP, obtaining a transfection efficiency of 15–20%, and GFP-expressing neurons were chosen to analyse tau localization. Importantly, overexpression of HDAC6 prevented Aβ-driven missorting of tau, which was polarized in the axon twofold more than in Aβ-treated neurons ( Fig. 5c,d ). Taken together, these results indicate that the inhibition of HDAC6 induced by Aβ is sufficient to increase acetylation of tau and to induce tau missorting in minor neurites, and that restoring of HDAC6 function might counteract Aβ phenotype. 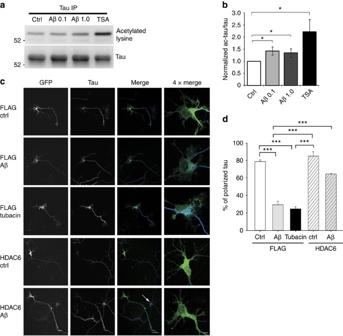Figure 5: Aβ increases acetylated tau and induces missorting of tau. (a) Representative immunoblot showing acetylation of tau immunoprecipitated from lysates of cortical neurons treated with either 0.05% DMSO (ctrl), 100 nM Aβ (Aβ 0.1), 1 μM Aβ (Aβ 1.0) or 100 nM TSA. Immunoprecipitated tau (bottom panel) was overlaid for acetylated lysine (top panel). (b) Quantification of the ratio between the protein level of acetylated tau and total tau in tau immunoprecipitates from neurons treated with either 0.05% DMSO (ctrl, 1.00±0.00,n=7), 100 nM Aβ (Aβ 0.1, 1.42±0.17,n=5), 1 μM Aβ (Aβ 1.0, 1.34±0.18,n=4) or 100 nM TSA (TSA, 2.22±0.52,n=7). Statistical significance determined by two-tailedt-test. Ctrl/Aβ 0.1:*P=0.012; ctrl/Aβ 1.0: *P=0.030; ctrl/TSA: *P=0.038. (c) Immunofluorescence analysis of tau localization (blue) in FLAG/GFP or HDAC6-FLAG/GFP-electroporated neurons (green), treated with either 0.05% DMSO (ctrl), 100 nM Aβ (Aβ) or 10 μM tubacin (tubacin), showing missorting of tau in minor neurites in the presence of Aβ, which is prevented by HDAC6 overexpression. Note, in the bottom panels showing neurons treated with Aβ, the presence of a non-electroporated neuron showing unpolarized tau staining (white arrow), and a neighbouring neuron overexpressing HDAC6 showing polarization of tau. Scale bar, 25 μm. Enlarged images of merged channels (far-right panels) showing minor neurites close to the cell body. Scale bar: 5 μm. (d) Quantification of the percentage of neurons showing polarized immunostaining of tau in axons, in neurons electroporated with FLAG/GFP and treated with either 0.05% DMSO (FLAG ctrl, 78.66±1.95,n=91), 100 nM Aβ (FLAG Aβ, 29.26±4.16,n=94), 10 μM tubacin (FLAG tubacin, 24.75±2.53,n=20) or electroporated with HDAC6-FLAG/GFP and treated with 0.05% DMSO (HDAC6 ctrl, 85.00±5.00,n=25) or 100 nM Aβ (HDAC6 Aβ, 64.32±0.68,n=31). Statistical significance determined by one-way ANOVA, ***P<0.001. Inbandd, data are expressed as mean±s.e.m. and as mean percentage±s.e.m., respectively. ANOVA, analysis of variance. Figure 5: Aβ increases acetylated tau and induces missorting of tau. ( a ) Representative immunoblot showing acetylation of tau immunoprecipitated from lysates of cortical neurons treated with either 0.05% DMSO (ctrl), 100 nM Aβ (Aβ 0.1), 1 μM Aβ (Aβ 1.0) or 100 nM TSA. Immunoprecipitated tau (bottom panel) was overlaid for acetylated lysine (top panel). ( b ) Quantification of the ratio between the protein level of acetylated tau and total tau in tau immunoprecipitates from neurons treated with either 0.05% DMSO (ctrl, 1.00±0.00, n =7), 100 nM Aβ (Aβ 0.1, 1.42±0.17, n =5), 1 μM Aβ (Aβ 1.0, 1.34±0.18, n =4) or 100 nM TSA (TSA, 2.22±0.52, n =7). Statistical significance determined by two-tailed t -test. Ctrl/Aβ 0.1:* P =0.012; ctrl/Aβ 1.0: * P =0.030; ctrl/TSA: * P =0.038. ( c ) Immunofluorescence analysis of tau localization (blue) in FLAG/GFP or HDAC6-FLAG/GFP-electroporated neurons (green), treated with either 0.05% DMSO (ctrl), 100 nM Aβ (Aβ) or 10 μM tubacin (tubacin), showing missorting of tau in minor neurites in the presence of Aβ, which is prevented by HDAC6 overexpression. Note, in the bottom panels showing neurons treated with Aβ, the presence of a non-electroporated neuron showing unpolarized tau staining (white arrow), and a neighbouring neuron overexpressing HDAC6 showing polarization of tau. Scale bar, 25 μm. Enlarged images of merged channels (far-right panels) showing minor neurites close to the cell body. Scale bar: 5 μm. ( d ) Quantification of the percentage of neurons showing polarized immunostaining of tau in axons, in neurons electroporated with FLAG/GFP and treated with either 0.05% DMSO (FLAG ctrl, 78.66±1.95, n =91), 100 nM Aβ (FLAG Aβ, 29.26±4.16, n =94), 10 μM tubacin (FLAG tubacin, 24.75±2.53, n =20) or electroporated with HDAC6-FLAG/GFP and treated with 0.05% DMSO (HDAC6 ctrl, 85.00±5.00, n =25) or 100 nM Aβ (HDAC6 Aβ, 64.32±0.68, n =31). Statistical significance determined by one-way ANOVA, *** P <0.001. In b and d , data are expressed as mean±s.e.m. and as mean percentage±s.e.m., respectively. ANOVA, analysis of variance. Full size image Aβ disrupts the integrity of the AIS In the maintenance of tau retrograde barrier, not only tau binding to MT is fundamental but also MT stability per se in the region overlapping with AIS [15] where EB3 is found enriched and less mobile [21] . To understand the possible mechanism of action of Aβ on axonal polarity in view of the observed missorting of tau-1, we measured the rate of movement of EB3 in the AIS ( Fig. 6a ). Kymographs of the EB3-GFP comets in the AIS regions of control neurons showed immobile EB3, whereas in Aβ-treated, as in tubacin-treated neurons, EB3 appeared more mobile ( Fig. 6b ). The speed of EB3 comets in the AIS of Aβ- and tubacin-treated neurons was increased by 45.3% and by 33.1%, respectively, in comparison with that of control ( Fig. 6c ; Supplementary Movies 1–3 ). Importantly, the destabilizing effect of Aβ on the MT in the AIS was no longer observed in neurons overexpressing HDAC6 ( Fig. 6b,c ; Supplementary Movies 4–5 ). As HDAC6 had been implicated in the maintenance of AIS [20] by its MT-binding activity, we investigated whether Aβ could modify the integrity of AIS by the analysis of ankG localization. Neurons exposed to Aβ and tubacin showed ankG staining no longer restricted to the AIS as in control neurons, but dispersed along the length of the axon ( Fig. 6d ). The length of ankG staining along the axon was increased by ∼ 30% and ∼ 40% in Aβ- and tubacin-treated neurons, respectively ( Fig. 6e ). AnkG dispersion was appreciable both in young neurons at 4 DIV and in neurons at later stage of development (14 DIV) ( Fig. 6d ; Supplementary Fig. 4b ). Given that previous studies provided direct evidence for a physiological role of ankG in the clustering of voltage-gated sodium channels into the axon initial segment [35] , we investigated whether Aβ treatment could interfere with the ability of the neuron to fire action potentials upon injection of current at the soma in whole-cell patch-clamp recordings. Examination of action potential profile revealed a marked increase of the spike threshold (defined by the membrane potential at which d V /d t of the spike crossed 15–20 mV ms −1 ) for Aβ-treated neurons compared with the control ones ( Fig. 6f–h ). Taken together, these results indicate that disruption of the AIS barrier by Aβ results in impaired action potential firing. 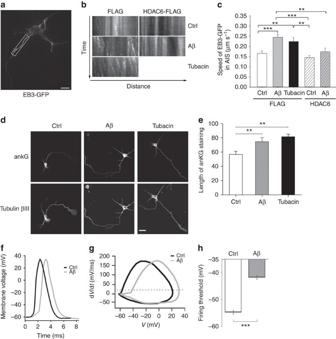Figure 6: Aβ disrupts the retrograde barrier of tau by destabilizing MT in the AIS and the integrity of AIS by mislocalizing ankG. (a) Confocal image of a neuron electroporated with HDAC6-FLAG and EB3-GFP, showing the region corresponding to the AIS (white rectangle). Scale bar, 10 μm. (b) Representative kymographs of the AIS of neurons co-electroporated with EB3-GFP and FLAG (left panels) or HDAC6-FLAG (right panels) and treated with 0.05% DMSO (ctrl), 100 nM Aβ (Aβ) or 10 μM tubacin (tubacin). The vertical arrow indicates the time (90 s) and the horizontal arrow indicates the direction from the cell body to the growth cone. (c) Quantification of the velocity of EB3-GFP comets in the AIS in neurons co-electroporated with EB3-GFP/FLAG (FLAG) and treated with either 0.05% DMSO (ctrl, 0.17±0.01,n=21), 100 nM Aβ for 1 h (Aβ, 0.24±0.01,n=11), 10 μM tubacin for 1 h (tubacin, 0.22±0.02,n=10) or electroporated with EB3-GFP/HDAC6-FLAG (HDAC6) and treated with 0.05% DMSO (ctrl, 0.14±0.01,n=11) or 100 nM Aβ for 1 h (Aβ, 0.17±0.02,n=12). Statistical significance determined by one-way ANOVA, ***P=0.001 (FLAG ctrl/FLAG Aβ), **P=0.019 (FLAG ctrl/FLAG tubacin), ***P<0.001 (HDAC6 ctrl/FLAG Aβ), **P=0.005 (HDAC6 ctrl/FLAG tubacin), **P=0.011 (FLAG Aβ/HDAC6 Aβ). (d) Immunofluorescence analysis of ankG and tubulin-βIII localization in neurons treated with either 0.05% DMSO (ctrl), 100 nM Aβ for 4 h (Aβ) or 10 μM tubacin (tubacin). Scale bar, 25 μm. (e) Quantification of the length of ankG staining along the axon of neurons treated with either 0.05% DMSO (ctrl, 56.78±4.41,n=52), 100 nM Aβ (Aβ, 74.49±5.94,n=68) or 10 μM tubacin (81.57±3.67,n=42). Statistical significance determined by one-way ANOVA, **P=0.006 (ctrl versus Aβ, ctrl versus tubacin). (f) Somatic current-clamp recording of a representative action potential evoked in neurons at 14 DIV treated for 4 h with 0.05% DMSO (black) or 100 nM Aβ (grey). (g) Phase plots of dV/dtversusVconstructed from recording as infin neurons treated for 4 h with 0.05% DMSO (black) or 100 nM Aβ (grey). (h) Quantification of the firing threshold of action potential in neurons treated with 0.05% DMSO (ctrl, −51.33±1.83,n=10) or Aβ (Aβ, −33.82±2.81,n=10). Statistical significance determined by two-tailedt-test, ***P<0.001. Inc,eandh, data are expressed as mean±s.e.m. ANOVA, analysis of variance. Figure 6: Aβ disrupts the retrograde barrier of tau by destabilizing MT in the AIS and the integrity of AIS by mislocalizing ankG. ( a ) Confocal image of a neuron electroporated with HDAC6-FLAG and EB3-GFP, showing the region corresponding to the AIS (white rectangle). Scale bar, 10 μm. ( b ) Representative kymographs of the AIS of neurons co-electroporated with EB3-GFP and FLAG (left panels) or HDAC6-FLAG (right panels) and treated with 0.05% DMSO (ctrl), 100 nM Aβ (Aβ) or 10 μM tubacin (tubacin). The vertical arrow indicates the time (90 s) and the horizontal arrow indicates the direction from the cell body to the growth cone. ( c ) Quantification of the velocity of EB3-GFP comets in the AIS in neurons co-electroporated with EB3-GFP/FLAG (FLAG) and treated with either 0.05% DMSO (ctrl, 0.17±0.01, n =21), 100 nM Aβ for 1 h (Aβ, 0.24±0.01, n =11), 10 μM tubacin for 1 h (tubacin, 0.22±0.02, n =10) or electroporated with EB3-GFP/HDAC6-FLAG (HDAC6) and treated with 0.05% DMSO (ctrl, 0.14±0.01, n =11) or 100 nM Aβ for 1 h (Aβ, 0.17±0.02, n =12). Statistical significance determined by one-way ANOVA, *** P =0.001 (FLAG ctrl/FLAG Aβ), ** P =0.019 (FLAG ctrl/FLAG tubacin), *** P <0.001 (HDAC6 ctrl/FLAG Aβ), ** P =0.005 (HDAC6 ctrl/FLAG tubacin), ** P =0.011 (FLAG Aβ/HDAC6 Aβ). ( d ) Immunofluorescence analysis of ankG and tubulin-βIII localization in neurons treated with either 0.05% DMSO (ctrl), 100 nM Aβ for 4 h (Aβ) or 10 μM tubacin (tubacin). Scale bar, 25 μm. ( e ) Quantification of the length of ankG staining along the axon of neurons treated with either 0.05% DMSO (ctrl, 56.78±4.41, n =52), 100 nM Aβ (Aβ, 74.49±5.94, n =68) or 10 μM tubacin (81.57±3.67, n =42). Statistical significance determined by one-way ANOVA, ** P =0.006 (ctrl versus Aβ, ctrl versus tubacin). ( f ) Somatic current-clamp recording of a representative action potential evoked in neurons at 14 DIV treated for 4 h with 0.05% DMSO (black) or 100 nM Aβ (grey). ( g ) Phase plots of d V /d t versus V constructed from recording as in f in neurons treated for 4 h with 0.05% DMSO (black) or 100 nM Aβ (grey). ( h ) Quantification of the firing threshold of action potential in neurons treated with 0.05% DMSO (ctrl, −51.33±1.83, n =10) or Aβ (Aβ, −33.82±2.81, n =10). Statistical significance determined by two-tailed t -test, *** P <0.001. In c , e and h , data are expressed as mean±s.e.m. ANOVA, analysis of variance. Full size image In this study, we provide evidence that submicromolar concentration of Aβ is able to alter actin and MT dynamics, via RhoA activation and inhibition of HDAC6, respectively. The altered cytoskeletal dynamics led to growth cone collapse, defect in axon elongation, and disruption of MT stability in the AIS, ultimately interfering with the maintenance of neuronal polarity. Using optical tweezers and microspheres coated with Aβ, we were able to study the local effect of extracellular Aβ, which induces growth cone collapse and neurite retraction in developing neurons. Our data suggest that soluble extracellular Aβ is sufficient in activating RhoA/ROCK pathway [36] , and also increases actin retrograde flow in a ROCK/myosin II-dependent manner. Indeed, inhibition of ROCK activity counteracted the effect of extracellular Aβ, preventing growth cone collapse and suggesting the possibility of a protective role of ROCK inhibitors in AD. The initial functional characterization of the members of the Ras superfamily of GTPases established actin cytoskeleton as their main target [37] , and later those observations were extended to reveal their function in the regulation of MT organization [38] . Growth cone movement is necessary for elongation and pathfinding of developing neurons. In ageing brain and in AD, an impairment of adult neurogenesis was found [39] that deepen the symptoms of neurodegenerative diseases due to loss of neurons. Therefore, an alteration in developmental processes that are fundamental for the correct migration of neurons might be at the basis of cell death in the areas of adult neurogenesis. These processes depend on coordinated action of microfilaments and MT [40] , prompting further investigation on the effect of Aβ on actin–MT crosstalk. To analyse MT dynamics, Aβ was added to the media of neurons, in which case the combined effect of Aβ both from the extracellular milieu and from inside the cells on its internalization was observed. We found that Aβ affected MT dynamics by inhibiting HDAC6, a deacetylase of tubulin and tau. While Aβ induced an increase in acetylation of MT, a marker of MT stability, the speeds of EB3 comets in neurons treated with Aβ, or with an HDAC6-specific inhibitor, tubacin, were faster than that in control neurons. In parallel, Aβ increased the rate of catastrophe/pause, a phenomenon that might arise from the contemporary action of Aβ on actin retrograde flow that impose a force counteracting MT growth [41] , indicating destabilization of MT as an overall effect, as MT undergo faster cycles of polymerization and depolymerization. The apparent contradiction between hyperacetylated MT and destabilized MT was explained by biochemical analysis of tubulin population that indicated that, in the presence of Aβ, the increase in acetylation was attributable more to tubulin heterodimers than to MT. Moreover, the heterodimeric fraction was further increased due to MT instability and to the inhibitory effect of Aβ on HDAC6. Increased myosin II-driven contractility together with MT instability in the axon would further exacerbate the tendency of the growth cone to collapse [40] , phenomenon that would affect growth cones motility in developing neurons or synapses stability in neuronal networks. Our data on the accumulation of ac-tub heterodimers might explain controversial data in previous reports on the level of tubulin acetylation. For example, AD pathology, which displays destabilized MT, was classically linked with a reduction of ac-tub [42] , whereas a more recent study on tau interaction with HDAC6 reported an increased level of ac-tub in AD samples [43] . Our results emphasize the importance of studying MT dynamics, besides tubulin post-translational modifications, in AD conditions when considering the use of HDAC6 inhibitors as a possible therapeutic approach for AD. Although the use of inhibitors that target various members of HDAC family, such as valporic acid, sodium butyrate and TSA, were demonstrated to be neuroprotective and to improve memory processes, most of the studies attributed the neuroprotective mechanism to HDAC 1–4 and Sirtuins, and not specifically to HDAC6 (ref. 44 ). Controversial data on protective or neurotoxic effect of HDAC6 are present in the literature. It was shown that tubastatin A, which specifically inhibits HDAC6, improved behavioural deficits, such as hyperactivity, fear conditioning and spatial navigation memory deficits in a transgenic mouse model of tauopathy [45] . A recent study correlated the amelioration of memory function induced by HDAC6 deletion in a model of AD, with the rescue in mitochondrial trafficking [46] . HDAC6 inhibition also improved the impaired mitochondrial transport in a model of Charcot–Marie–Tooth disease [47] , and nonspecific HDAC inhibitors, such as suberoylanilide hydroxamic acid and TSA, application alleviates the impaired axonal transport of vesicles by enhancing the interaction between kinesin-1 and MT in a mouse model of Huntington’s disease [48] . On the other hand, another group showed that genetic depletion of HDAC6 did not modify the progression of Hungtinton’s disease [49] . It was also shown that phosphorylation of HDAC6, activating its deacetylase activity, promotes proper aggresome formation and protects from toxicity [50] . Indeed, HDAC6 inhibition would impair the removal of aggregated protein by retrograde transport to autophagosomes and lysosomes as it was shown that tubacin treatment decreased the recruitment of Atg/LC3, a crucial component of autophagic transport [51] , and that HDAC6 expression rescued neurodegeneration in a model of spinal and bulbar muscular atrophy [52] . HDAC6 has been shown also to protect dopaminergic neurons from alpha-synuclein-induced toxicity [53] . For what concerns axonal pathology, MT stability must be regulated at an optimal level to allow axon and dendrites development in neuritogenesis, and it has been demonstrated that HDAC6 is required to provide efficient MT deacetylation [54] . Consistently, it has been shown that silencing of HDAC6 reduced neurite outgrowth and that its retransfection was able to revert to the normal phenotype [55] . It is thus critical to consider the deacetylase isoforms, and the specific function defective in the diseases, to evaluate HDACs or HDACs inhibitors for therapeutic intervention. Acetylation occurs on lysine, the same amino acid on which ubiquitination for protein degradation takes place. Further experiments would be needed to study if acetylated heterodimeric tubulin can still be ubiquitinated by ubiquitin ligases [56] . Tau interacts and is deacetylated by HDAC6 (ref. 57 ), in fact TSA treatment leads to dramatic accumulation of ac-tau, and ac-tau was found in NFTs in various neurodegenerative diseases [16] , [17] . Phosphorylation of tau, a modification of tau that underlies tau-mediated degeneration, and that was shown to impair synaptic function at preclinical stages of disease [58] , has been associated with this acetylation state. Indeed, tau acetylation was shown to prevent the degradation of phosphorylated tau [17] . Both forms have impaired MT binding, which results in further MT instability [16] . A recent study in oligodendrocytes showed that inhibition of HDAC6 caused an increase in hyperphosphorylated tau that disrupts its interaction with MT [59] . Interestingly, a recent report showed that mutant tau associated with tauopathies is sequestered by its binding to heterodimeric tubulin, suggesting a role of unpolymerized tubulin in AD and other tau pathologies [60] . Moreover, overexpression of tau was shown to increase ac-tub in fibroblasts [61] , which may be explained by tau-driven inhibition of HDAC6 (ref. 43 ). This gives rise to the possibility that polarized cells, such as neurons, which express high level of tau and ac-tub, may be more susceptible to changes in tau and/or tubulin levels induced by Aβ in comparison with other cell types. It is noteworthy that both substrates of HDAC6, ac-tub and tau, are enriched in axons, suggesting a role of HDAC6 in neuronal polarity. Here we provide evidence that maintenance of polarized axonal identity is disrupted by Aβ in an HDAC6-dependent manner. Importantly, overexpression of HDAC6 was sufficient to prevent the effect of Aβ, and, together, with a decrease in ac-tub and tau, a function of HDAC6 as a MAP [20] , [22] may be implicated in the maintenance of stabilized MT in the AIS. Neuron polarization consists of morphological polarization that involve preferential elongation of the axon; sorting of proteins in different compartments; and functional polarization, in which the AIS barrier is also involved. It is a very complex phenomenon that requires local destabilization of actin [62] and local stabilization of MTs [63] . RhoA activation is known to decrease actin turnover, stabilizing actin, and thus participating in axon retraction [64] . Moreover, human mutant tau has the ability to bind and bundle F-actin in vitro [65] . Aβ-driven actin stabilization and MT destabilization are therefore both possibly hampering neuronal elongation and polarization, not excluding the possibility of a mechanistic link mediated by other players. Finally, we showed that ankG and sodium channels are dispersed along the axon on exposure to Aβ. Consistently, a recent report showed defective filtering at the axon initial segment in cultured neurons from an AD mouse model [66] . In conclusion, as summarized in the model shown in Fig. 7 , our study demonstrates that extracellular Aβ and intracellular Aβ target RhoA and HDAC6, respectively, altering actin and MT dynamics. The activity of Aβ on its targets leads to increased actin retrograde flow, instability of MT and hyperacetylation and missorting of tau. The combined effects on cytoskeletal dynamics and acetylation levels induce loss of AIS integrity and impairment in action potential firing, implicating RhoA and HDAC6 in the interplay between Aβ and tau in AD. 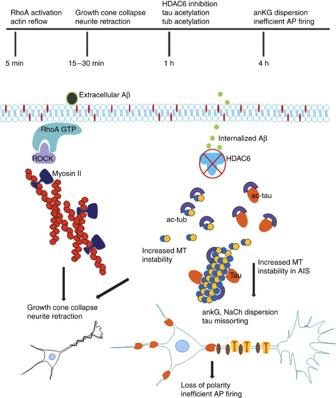Figure 7: Model of Aβ’s mechanisms of action. The upper part illustrates a hypothetical time course showing short- and long-term effects of Aβ in our experimental conditions. The lower part shows a cartoon of the combined effects of extracellular and intracellular Aβ. Extracellular Aβ, which is kept in contact with the cell surface, activates RhoA and its downstream targets ROCK and myosin II, increasing actin retrograde flow. Internalized soluble Aβ inhibits HDAC6 inducing an increase in the acetylation of tubulin heterodimers. In parallel, tau is also hyperacetylated due to HDAC6 inhibition, and MT instability is favoured. The alterations of the dynamics of both cytoskeletal elements induce growth cone collapse and neurite retraction. MT instability in the AIS in particular leads to dispersion of ankG (brown ovals) and of Na+channels (yellow channels) outside the AIS, and to missorting of tau in dendrites, with ensuing loss of neuronal polarity and inefficient AP firing. Figure 7: Model of Aβ’s mechanisms of action. The upper part illustrates a hypothetical time course showing short- and long-term effects of Aβ in our experimental conditions. The lower part shows a cartoon of the combined effects of extracellular and intracellular Aβ. Extracellular Aβ, which is kept in contact with the cell surface, activates RhoA and its downstream targets ROCK and myosin II, increasing actin retrograde flow. Internalized soluble Aβ inhibits HDAC6 inducing an increase in the acetylation of tubulin heterodimers. In parallel, tau is also hyperacetylated due to HDAC6 inhibition, and MT instability is favoured. The alterations of the dynamics of both cytoskeletal elements induce growth cone collapse and neurite retraction. MT instability in the AIS in particular leads to dispersion of ankG (brown ovals) and of Na + channels (yellow channels) outside the AIS, and to missorting of tau in dendrites, with ensuing loss of neuronal polarity and inefficient AP firing. Full size image Peptides β-Amyloid (1–42), HiLyte Fluor 488-labelled β-amyloid (1–42) and scrambled β-amyloid (1–42) were purchased from Anaspec, Inc. (Fremont, CA, USA). The peptides were solubilized in 100%dimethylsulphoxide, aliquoted and kept at −80 °C. Reagents Blebbistatin, TSA, tubacin and taxol were purchased from Sigma-Aldrich (St Louis, MO, USA). Y27632 was purchased from Millipore Corporation (Billerica, MA, USA). Expression plasmids pRaichu-1298 × was a kind gift from Professor Michiyuki Matsuda (Kyoto University, Kyoto, Japan); pEGFP-N1-LifeAct was a kind gift from Dr Giorgio Scita (IFOM, Milan, Italy); pEGFP-N1 was purchased from Clonetech Laboratories, Inc. (Mountain View, CA, USA); pCMV-AC-GFP-EB3-GFP was purchased from Origene Technologies, Inc. (Rockville, MD, USA); pCDNA3.1-HDAC6-FLAG-was purchased from Addgene, Inc. (Cambridge, MA, USA); and pCMV-FLAG-3 × was purchased from Sigma-Aldrich. Antibodies The antibodies used were as following: monoclonal anti-ac-tub and anti-pan-Na + channel (Sigma-Aldrich); anti-tubulin-βIII, anti-MAP2 and anti-Aβ 6E10 (Covance, Princeton, NJ, USA); anti-acetylated lysine (Cell Signaling Technology Inc., Danvers, MA, USA); anti-ankG (Life Technologies, Paisley, UK); anti-tau: Tau-1 and Tau-5 (Merck Millipore, Billerica, MA, USA); and polyclonal anti-tubulin-βIII (Sigma-Aldrich). All antibodies were used at a dilution of 1:1,000 for immunoblotting experiments and of 1:100 for immunoistochemistry experiments. Neuronal culture All experiments were performed in accordance with Italian Ministry of Health. Primary cultures were obtained from hippocampi or cortices derived from embryonic day 18 C57BL6J mice (Harlan Laboratories Inc., Indianapolis, IN, USA). Embryos were removed and dissected under sterile conditions. Cortices and hippocampi were dissociated by enzymatic digestion in 0.125% trypsin-EDTA (Life Technologies) for 30 min at 37 o C and cortices were further treated with 0.25 mg ml −1 DNase in Hank’s balanced saline solution (Life Technologies)/2 mM calcium chloride (Sigma-Aldrich) for 30 min at 37 °C. Trypsin activity was blocked by adding complete medium, which consists of Neurobasal Media (Life Technologies) supplemented with 2% B27 (Life Technologies), 2 mM GlutaMax (Life Technologies), 100 U ml −1 penicillin–streptomycin (Life Technologies) and 10% fetal bovine serum (FBS; Life Technologies). After trypsinization, hippocampi were rinsed in complete medium without FBS, dissociated with a plastic pipette, and 20,000–40,000 hippocampal neurons were plated at a concentration of 0.20–1 × 10 5 cells per millilitre on 18-mm diameter coverslips precoated with 0.1 mg ml −1 poly- D -lysine (Sigma-Aldrich). After trypsinization, cortices were rinsed in the complete media without FBS, dissociated with a plastic pipette and centrifuged at 1,500 g for 7 min, and 2 × 10 6 cortical neurons were plated 60-mm diameter Petri dishes precoated with 0.01 mg ml −1 poly- D -lysine (Sigma-Aldrich). Atomic force microscopy AFM imaging was performed employing a Nanowizard II (JPK instruments, Germany) in intermittent contact mode, in air. Single-beam uncoated silicon cantilevers (OMCL-AC160TS-W, Olympus, Japan) with typical resonance frequency of 300 kHz were used. The nominal tip radius of curvature of the tip is 10 nm. Fifteen microlitres aliquots of 12 μM Aβ incubated for different times in Neurobasal were deposited on freshly cleaved mica substrates and allowed to adhere for 10 min, before washing with water and drying under a gentle N 2 stream. Immunocytochemistry and confocal microscopy Primary hippocampal neurons cultured on coverslips were fixed in 4% paraformaldehyde/30% glycerol in PBS for 7 min. The neurons immunostained for ankG were treated with cold 100% methanol for 5 min at −20 °C after fixation. The coverslips were washed in PBS four times and were incubated with primary antibodies. After four washes in 20 mM phosphate buffer with 0.5 M NaCl, fluorescently conjugated secondary antibodies in 5% normal goat serum/0.1% Triton in PBS were added to the coverslips. The coverslips were washed in 20 mM phosphate buffer with 0.5 M NaCl four times, once in PBS and dipped in distilled water before being mounted in ProLong Gold Antifade Reagent (Life Technologies). Confocal images were acquired on a Leica TCS SP5 microscope using a 63 × objective (Leica Microsystems, Wetzlar, Germany). Axonal length Primary hippocampal neurons plated on 18-mm diameter coverslips were incubated with 1 μM Aβ for 1 h. The neurons were immunostained with anti-tubulin-βIII as described above. All neurites were traced using NeuronJ plug-in in ImageJ, and the length of the longest neurite, considered as axon, was measured using ImageJ. Electroporation of primary hippocampal neurons Neurons (1 × 10 6 ) were electroporated with 1 μg of DNA using P3 Primary Cell 4D-Nucleofector Kit and the pulse code CU133 on the 4D-Nucleofector System (Lonza Group Ltd, Basel, Switzerland). Coating of microspheres with beta-amyloid peptides Three micrograms of carboxyl polymer microspheres of 4.08 μm diameter (Bangs Laboratories Inc., Fishers, IN, USA) were washed and resuspended in coupling buffer from Poly-Link Coupling Kit for (Polysciences Inc., Warrington, PA, USA) containing 0.022 mg μl −1 of 1,3-propanediamine, N ′-(ethylcarbonimidoyl)- N , N -dimethyl-monohydrochloride (EDAC) for 2 h at room temperature. EDAC solution was removed by centrifugation at 1,000 g for 10 min, the microspheres were washed in the coupling buffer without EDAC. The activated microspheres were resuspended in 10 mM phosphate buffer at pH 7.4 containing 1 μg μl −1 β-amyloid (1–42), HiLyte Fluor 488-labelled β-amyloid (1–42) or scrambled-β-amyloid (1–42) (Anaspec Inc.) incubated at 4 o C overnight. Excess unbound peptide was removed by centrifugation at 1,000 g for 5 min at 4 °C and the microspheres were resuspended in 10 mM phosphate buffer to the concentration of 0.06 μg μl −1 . Microspheres coated with the desired peptide were resuspended in the conditioned medium from the neuronal culture at a concentration of 0.04 μg μl −1 , and a total of 0.4 μg was added to the neuron dish placed in the optical setup equipped with an incubator maintained at 35 °C with 5% CO 2 balanced with air [67] . Force spectroscopy measurements We applied interferometric tracking of a functionalized microsphere held in an optical trap and brought in contact with the neck of the axonal growth cone of a mouse neuron. The optical system to perform long-term force spectroscopy measurements was previously described in detail [25] . Briefly, it consists of a modified upright microscope integrating an optical tweezers system working in force-clamp condition (with force equal to zero). The position of the bead with respect to the centre of the trap ( x QPD , y QPD and z QPD ) is measured through a QPD. During the interaction with the cell, the system is operated in force-clamp with a 0 pN set point. To keep the bead in the centre of the trap, the QPD signal is fed back to a proportional-integral stage driving the coarse motion of a three axis piezo stage (PIEZO) in space (S x , S y and S z ). QPD and PIEZO signals were sampled independently and simultaneously at a 2 kHz acquisition rate, while bright-field images were acquired at 1 Hz frame rate and synchronized in time with the data. For every experiment, the bead was positioned in contact with the neck of the growth cone, the region connecting the growth cone with the axon shaft. Supplementary Figure 2a shows a typical example of a growth cone rearranging its shape around the trapped microsphere, while the corresponding spatial trajectory (S x , S y and S z ) and QPD signals (forces) are reported in Supplementary Fig. 2b . A complementary representation of the same experiment is reported in Supplementary Fig. 2c in which the shift of the microsphere on the membrane apical surface is shown by the cyan line, and the random forces acting on the microsphere are represented as vector field (coloured arrows). To obtain this representation, average force acting on the microsphere was calculated by vector-averaging the displacement from the trap centre over a time window of 1 s, multiplied by the calibrated trapping stiffness (that was kept constant along the whole experiment). Independent information can be obtained by analysis of the QPD and PIEZO signals. The QPD traces encode higher frequencies that are associated with the Brownian motion of the cell-adhered probe (in x , y and z directions). When the bond between the cell and the bead tightens, the average motion of the bead is reduced, and is indicated by a measurable drop in the variance of the signal, var QPD ( Supplementary Fig. 2d ). The variance of the QPD motion was computed as the total variance of x QPD , y QPD and z QPD traces on a time-shifted window of 6,000 points, with half-time window (3,000 points) overlap (the variance is computed each 1.5 s). The decrease of the variance of cell-adhered bead Δvar=var QPD, t =0 −var QPD, t =end ( t =end, indicate the last acquired time point) was calculated with respect to the value of the first second of recording and normalized to the total duration of the experiment: Δvar/Δ t (typical duration of an experimental session is 45 min). Alongside, PIEZO signals encode lower frequency information associated with the overall motion of the probe on the apical surface of the growth cone, and thus on the local remodelling of the leading edge of the cell, through cytoskeleton and molecular motor dynamics [68] . The vertical position of the bead, S z (see an example in Supplementary Fig. 2e ), was taken as a direct measure of the growth cone state, and its shrinking on local application of coated microsphere was quantified in terms of the total vertical displacement: ΔS z = z PIEZO, t =0 − z PIEZO, t =end . Moreover, the in-plane velocity of the bead was calculated by interpolation of the spatial trajectory (S x and S y ) over a time interval of 100 ms (that is, 200 points window) and the modulus V =( V S x ) 2 +( V S y ) 2 was taken as a reference of the speed of the bead on the cell surface. FRET analysis Microsphere coated as described above was attached to a neurite of 3 DIV hippocampal neurons electroporated with pRaichu-1298 × and time-lapse images were taken every 20 s for a total of 30 min. FRET probes were excited with a TTL modulated 405-nm laser source (1-s light pulse duration), and the emitted fluorescence light was collected and separated through a dichroic mirror and sent to two synchronized charge-coupled devices (CCDs; acquiring the distinct donor–acceptors signals). The CCDs integrated the emitted photons during the 20 s time frame period. Therefore, we could reduce the light exposure, and avoid the unwanted photobleaching of donor–acceptor dyes. To quantify the FRET efficiency, we register the two acquired stack trough image cross-correlation (Huygens software), we subtracted the background signals and detect the cell area trough image segmentation (ImageJ). Then, we compute the ratio imaging on the identified cell region of interest in the field of view. FRET ratio where normalized to the baseline value prestimulation. To compute the FRET efficiency increase, we calculate the averaged FRET value on the stimulated axon region of interest for each time frame. Live imaging of actin retrograde flow Hippocampal neurons from embryonic day 18 mouse embryos prepared as described above were plated onto a glass bottom dish (MatTek Corporation, Ashland, MA, USA) at 2,000 neurons per millimetre. A coated microsphere was optically driven in contact with the neck of a growth cone, and a time-lapse movie of LifeAct-GFP was acquired. Fluorochromes were excited with a TTL modulated (200-ms light pulse duration) 473-nm laser source (TECBL-15 G-473-TTL-FC, World Star Tech. Inc., USA), and the emitted fluorescence was integrated during the 1-s time frame period through the CCD (V887 ECS UVB EMCCD, Andor, Italy). Kymographs of LifeAct-GFP time-lapse movies were constructed using MultipleKymograph plug-in of ImageJ. Live imaging and EB3-GFP tracking Time-lapse images of GFP comets in mouse hippocampal neurons electroporated with EB3-GFP were taken in total internal reflection mode set at 250 nm on Leica TCS SP5 microscope with a 100 × objective (Leica Microsystems, Wetzlar, Germany) at 1 frame per second for 90 s. For MT dynamics neurons at 3 DIV were used, whereas neurons at 5 DIV were used for MT dynamics in the AIS. The speed of the GFP comets was analysed using the object analyser in Huygens Professionals v.3.7 (Scientific Volume Imaging B.V., Hilversum, The Netherlands). Kymographs of EB3-GFP time-lapse movies were constructed using MultipleKymograph plug-in of ImageJ. Number of catastrophes/pause per MT were counted as gaps in the EB3-GFP lines in the kymographs, which were created from the corresponding time-lapse movies using Image J as described above. In vitro assay of HDAC6 catalytic activity Catalytic activity of HDAC6 was assayed in the presence of 0.05% DMSO, 50 nM TSA, 100 nM Aβ or 1 μM Aβ using Fluor-de-Lys HDAC6 fluorometric drug discovery kit (Enzo Life Sciences, Inc., Farmingdale, NY, USA) according to the manufacturer’s instructions. Separation of tubulin and MTs Cortical neurons (2 × 10 6 ) were fixed with 4% paraformaldehyde in PBS for 1 min. After fixation neurons were homogenized in 200 μl of PBS, with 0.1% Triton X-100, protease inhibitor cocktail (Roche, Basel, Switzerland) and phosphatase inhibitor cocktails 2 and 3 (Sigma-Aldrich) by passing through needle of 28 G × 1/2 in (BD, Franklin Lakes, NJ, USA) for five passages at room temperature. The homogenates were centrifuged at 1,000 g to remove cell debris and the proteins were separated by 7% SDS–polyacrylamide gel electrophoresis (SDS–PAGE). Immunoblotting Following 10% SDS–PAGE, proteins were transferred onto nitrocellulose membrane, blocked in 5% milk/TBS/Tween 0.05% for 1 h at room temperature and incubated with primary antibodies for 2 h at room temperature. The membranes were washed four times for a total of 30 min in TBS/Tween 0.05% and incubated with horseradish peroxidase-conjugated secondary antibody for 1 h at room temperature. The membranes were washed four times for a total of 30 min in TBS/Tween 0.05%, overlayed with Amersham ECL Western Blotting Detection Reagent (GE Healthcare Life Sciences, Freiburg, Germany) and imaged for chemiluminescence using ImageQuant LAS 500 (GE Healthcare Life Sciences). Permeabilization before immunocytochemistry Primary hippocampal neurons cultured on coverslips were gently covered with MSB with 0.1% Triton X-100 for 10 s at room temperature before fixation in 4% paraformaldehyde/4% sucrose in PBS. Following the fixation, the neurons were immunostained as described above. Tau immunoprecipitation Cortical neurons (2 × 10 6 ) were homogenized in 100 μl of MSB/150 mM NaCl/0.5% Triton-X with protease inhibitor cocktail (Roche) and phosphatase inhibitor cocktails 2 and 3 (Sigma-Aldrich) by passing through needle of 28 G × 1/2 in (BD) for 10 passages at room temperature and left on ice for 30 min. Twenty microgram of total protein was incubated with 1 μg of tau-1 antibody for 2 h at 4 °C. Antibody-bound fractions were pulled down with Protein G-Sepharose 4B (GE Healthcare Life Sciences), washed with MSB containing 0.1% Triton-X twice before eluting in the laemmli buffer and boiled at 100 °C for 5 min. The immunoprecipitates were separated by SDS–PAGE and immnoblotted using as described above. Electrophysiological recordings Action potentials were recorded in the whole-cell configuration of the patch-clamp technique. The extracellular recording solution (145 mM NaCl/2 mM KCl/2 mM MgCl 2 /1 mM CaCl 2 /10 mM glucose/10 mM HEPES, pH 7.4), patch pipettes pulled from borosilicate glass capillaries (Hilgenberg, Malsfeld, Germany) had a 4–5 MΩ resistance when filled with intracellular recording solution (130 mM K-gluconate/5 mM KCl/5 mM sucrose/1 mM EGTA/10 mM HEPES/4 mM Mg-ATP, 300 mOsm and pH 7.2 with KOH). Cells were current clamped at about −65 mV and the action potentials evoked were acquired using Clampex 10.0 software (Molecular Devices, Sunnyvale, CA, USA). During the experiments, the stability of the patch was checked by continuously monitoring the series resistance: cells exhibiting 10–15% changes were excluded from the analysis. Currents were sampled at 10 kHz and digitally filtered at 3 kHz using the 700B Axopatch amplifier (Molecular Devices). During the experiments, neurons were continuously perfused at 12 ml h −1 with the extracellular recording solution. Statistical analysis Two-tailed tests were performed using SigmaPlot 12.0 (Systat Software, Inc., San Jose, CA, USA) for comparison of two groups and expressed as mean values±s.e.m. For all pair-wise multiple comparison procedure, Holm–Sidak method was used for one-way analysis of variance using SigmaPlot 12.0 (Systat Software), and the data were expressed as mean values±s.e.m. P -values <0.05 were considered to be statistically significant. The power of performed test with alpha ( π ) for the statistical analysis and when the t -tests were used, the t -values, the degrees of freedom (df) are also included as follows: Fig. 1a : t =6.170, df=291, π =0.050:1.000; Fig. 1e : ctrl versus Aβ: t =5.450, df=10, π =0.050:0.999; Aβ versus Aβ+Y27632: t =−2.547, df=8, π =0.050:0.536; Aβ versus Aβ+blebb: t =−3.546, df=7, π =0.050:0.849; Fig. 2a : π =0.050:0.711; Fig. 2b : π =0.050:0.966; Fig. 2f : t =−3.837, df=14, π =0.050:0.944; Fig. 2i : t =−3.359, df=86, π =0.050:0.906; Fig. 3b : π =0.050:0.854; Fig. 3c : π =0.050:0.961; Fig. 4b : π =0.050:0.486; Fig. 4c : π =0.050:1.000; Fig. 4e : MT: π =0.050:1.000, monomers: π =0.050:0.962; Fig. 4f : t =−3.549, df=59, π =0.050:0.935; Fig. 5b : ctrl versus Aβ0.1: t =−3.053, df=10, π =0.050:0.747; ctrl versus Aβ1.0: t =2.573, df=9, π =0.050:0.559; ctrl versus TSA: t =−1.218, df=12, π =0.050:0.482; Fig. 5d : π =0.050:1.000; Fig. 6c : π =0.050:0.994; Fig. 6e : π =0.050:0.744; Fig. 6h : ctrl versus Aβ: t =−5.210, df=18, π =0.050:0.999. How to cite this article: Tsushima, H. et al. HDAC6 and RhoA are novel players in Abeta-driven disruption of neuronal polarity. Nat. Commun. 6:7781 doi: 10.1038/ncomms8781 (2015).